Origin of the unique ventilatory apparatus of turtles The turtle body plan differs markedly from that of other vertebrates and serves as a model system for studying structural and developmental evolution. Incorporation of the ribs into the turtle shell negates the costal movements that effect lung ventilation in other air-breathing amniotes. Instead, turtles have a unique abdominal-muscle-based ventilatory apparatus whose evolutionary origins have remained mysterious. Here we show through broadly comparative anatomical and histological analyses that an early member of the turtle stem lineage has several turtle-specific ventilation characters: rigid ribcage, inferred loss of intercostal muscles and osteological correlates of the primary expiratory muscle. Our results suggest that the ventilation mechanism of turtles evolved through a division of labour between the ribs and muscles of the trunk in which the abdominal muscles took on the primary ventilatory function, whereas the broadened ribs became the primary means of stabilizing the trunk. These changes occurred approximately 50 million years before the evolution of the fully ossified shell. Extant amniotes (the clade comprising mammals, turtles, birds, crocodilians and lepidosaurs) ventilate their lungs using a diversity of mechanisms ( Fig. 1a ). The most common of these solutions involves expansion and contraction of the ribcage effected by the intercostal muscles, either primarily, as in lepidosaurs (squamates and tuataras) or to supplement previously accessory structures that eventually became primary (for example, mammalian diaphragm) [1] , [2] . Costal ventilation is impossible in turtles because their intercostal muscles are lost during embryogenesis [3] and their ribs are bound in a typically rigid shell [4] . Instead, turtles employ a unique apparatus mainly involving two paired, antagonistic abdominal (hypaxial) muscles: M. transversus (including the ‘M. diaphragmaticus’ of others [5] , [6] ; see results) and M. obliquus abdominis [6] , [7] ( Figs 1b,c , 2 ). The M. transversus includes two bellies that originate separately from the cranial (M. t. thoracis) and caudal (M. t. abdominis) portions of the shell and run towards one another ventrally before merging via a tendinous aponeurosis. The muscle thus serves as a sling-like functional unit that largely embraces the coelomic cavity and thereby the viscera. Contraction of the M. transversus initiates expiration by pressing the ventrally positioned viscera against the dorsally positioned lungs, which increases intrapulmonary pressure [7] , [8] . Inspiration is effected by the posteriorly positioned M. obliquus abdominis, which when relaxed exhibits a concave, dome-like shape in the caudal flank region between the hind limbs and the bridge of the shell ( Fig. 1b,c ). Contraction and flattening of the M. obliquus abdominis initiates inspiration by pulling the M. transversus and underlying peritoneum caudoventrally, which decreases intrapulmonary pressure [6] , [7] ( Fig. 1b,c ). 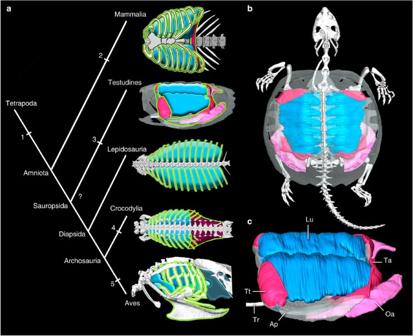Figure 1: Evolution of ventilatory mechanisms in Amniota. (a) Plesiomorphic costal ventilation (1) is employed in Lepidosauria (for example,V. exanthematicus) and in taxa with a diaphragm (Mammalia:Hylobatessp.; 2), hepatic piston (Crocodylia:A. mississippiensis; 4) and sternal pump (G. domesticus; 5), but not in turtles (Testudines:C. serpentina), which have a unique abdominal muscle-based mechanism (3). Phylogeny is derived from morphology4,17,43,44. Molecular results switch the positions of Testudines and Lepidosauria45,46,47but do not affect our inferences regarding the evolution of lung ventilation in turtles. (b,c) Digital reconstruction of the skeleton, lungs and hypaxial muscles ofC. serpentina(b, dorsal view;cdorsolateral view). Ap, tendinous aponeurosis; Lu, lung; Oa, M. obliquus abdominis; Ta, M. transversus abdominis; Tr, trachea; Tt, M. transversus thoracis. Figure 1: Evolution of ventilatory mechanisms in Amniota. ( a ) Plesiomorphic costal ventilation (1) is employed in Lepidosauria (for example, V. exanthematicus ) and in taxa with a diaphragm (Mammalia: Hylobates sp. ; 2), hepatic piston (Crocodylia: A. mississippiensis ; 4) and sternal pump ( G. domesticus ; 5), but not in turtles (Testudines: C. serpentina ), which have a unique abdominal muscle-based mechanism (3). Phylogeny is derived from morphology [4] , [17] , [43] , [44] . Molecular results switch the positions of Testudines and Lepidosauria [45] , [46] , [47] but do not affect our inferences regarding the evolution of lung ventilation in turtles. ( b , c ) Digital reconstruction of the skeleton, lungs and hypaxial muscles of C. serpentina ( b , dorsal view; c dorsolateral view). Ap, tendinous aponeurosis; Lu, lung; Oa, M. obliquus abdominis; Ta, M. transversus abdominis; Tr, trachea; Tt, M. transversus thoracis. 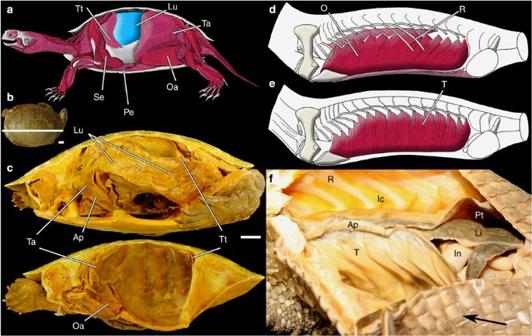Figure 2: Comparison of the deep hypaxial muscles in turtles and tuataraSphenodon punctatus. (a) Diagrammatic image of a European pond turtle,Emys orbicularis(Emydidae), illustrating the cup-like form of the caudal M. obliquus abdominis (Oa) and the cranial M. serratus (Se). The M. transversus thoracis (Tt) originates on dorsal rib three and encloses the cranial portion of the lung (Lu). The M. transversus abdominis (Ta) originates from the dorsal ribs five to eight and inserts into a tendinous aponeurosis ventrally. Redrawn from Bojanus5. (b)Emydura subglobosa(Chelidae) (USNM 574459) with white line showing where the shell was cut. Scale bar, 2 cm. (c) Lateral view with the shell cut longitudinally (top), showing the major respiratory muscles, lungs and viscera (except the liver, which has been removed)in situ. The M. transversus thoracis (Tt) originates on dorsal rib three and inserts into a tendinous aponeurosis (Ap) that lies superficial to the peritoneum. Right portion of the shell (bottom) showing the origination sites for the major respiratory muscles. The M. transversus abdominis (Ta) originates on dorsal rib five and inserts into a tendinous aponeurosis ventrally. Scale bar, 2 cm. (d) InS. punctatus, the M. obliquus (O) forms a continuous sheath between the shoulder and pelvic girdle and originates from tendinous sheaths attached to each dorsal rib (R). (e) The M. transversus (T) ofS. punctatusis the deepest layer of the hypaxial body wall muscles, and is situated just superficial to the peritoneum. It extends between the shoulder and pelvic girdles and originates from the ventral surface of each boney rib just dorsal to the cartilaginous uncinate processes. The fibres of the three cranial-most bundles insert on the dorsolateral margin of the sternum, whereas those of the remaining bundles insert into a midventral tendinous aponeurosis (Ap).dandeare modified after Maurer32. (f) Ventrolateral view from the anatomical right side of the trunk inS. punctatus(ZSM 1318/2006; snout-vent length=192 mm) showing the M. transversus (T) inserting ventrally into a tendinous aponeurosis (Ap). The peritoneum is opened in the abdominal region revealing the liver (Li) and intestine (In). Ic: M. intercostalis. Arrow points cranially. Full size image Figure 2: Comparison of the deep hypaxial muscles in turtles and tuatara Sphenodon punctatus. ( a ) Diagrammatic image of a European pond turtle, Emys orbicularis (Emydidae), illustrating the cup-like form of the caudal M. obliquus abdominis (Oa) and the cranial M. serratus (Se). The M. transversus thoracis (Tt) originates on dorsal rib three and encloses the cranial portion of the lung (Lu). The M. transversus abdominis (Ta) originates from the dorsal ribs five to eight and inserts into a tendinous aponeurosis ventrally. Redrawn from Bojanus [5] . ( b ) Emydura subglobosa (Chelidae) (USNM 574459) with white line showing where the shell was cut. Scale bar, 2 cm. ( c ) Lateral view with the shell cut longitudinally (top), showing the major respiratory muscles, lungs and viscera (except the liver, which has been removed) in situ . The M. transversus thoracis (Tt) originates on dorsal rib three and inserts into a tendinous aponeurosis (Ap) that lies superficial to the peritoneum. Right portion of the shell (bottom) showing the origination sites for the major respiratory muscles. The M. transversus abdominis (Ta) originates on dorsal rib five and inserts into a tendinous aponeurosis ventrally. Scale bar, 2 cm. ( d ) In S. punctatus , the M. obliquus (O) forms a continuous sheath between the shoulder and pelvic girdle and originates from tendinous sheaths attached to each dorsal rib (R). ( e ) The M. transversus (T) of S. punctatus is the deepest layer of the hypaxial body wall muscles, and is situated just superficial to the peritoneum. It extends between the shoulder and pelvic girdles and originates from the ventral surface of each boney rib just dorsal to the cartilaginous uncinate processes. The fibres of the three cranial-most bundles insert on the dorsolateral margin of the sternum, whereas those of the remaining bundles insert into a midventral tendinous aponeurosis (Ap). d and e are modified after Maurer [32] . ( f ) Ventrolateral view from the anatomical right side of the trunk in S. punctatus (ZSM 1318/2006; snout-vent length=192 mm) showing the M. transversus (T) inserting ventrally into a tendinous aponeurosis (Ap). The peritoneum is opened in the abdominal region revealing the liver (Li) and intestine (In). Ic: M. intercostalis. Arrow points cranially. Full size image In most amniotes, the dorsal ribs and hypaxial muscles serve the dual function of ventilating the lungs and stabilizing the trunk against torsional forces generated during locomotion [8] , [9] . Turtles have divided these functions, with the dorsal ribs only stabilizing the trunk and the hypaxial muscles exclusively effecting ventilation [10] , [11] , [12] ; however, it is unclear how and when such a division could have evolved. The need to maintain respiratory function and the ancestral role of the dorsal ribs in lung ventilation dictate that either the unique abdominal muscle apparatus or an alternative ventilatory mechanism was in place in the turtle stem lineage before the fusion of the ribs [11] , [12] . To understand the origin of the pulmonary ventilatory mechanism of turtles, we homologize the hypaxial muscles used in extant turtle respiration with those found in other tetrapods. We then analyse the trunk anatomy of two early stem turtles, Odontochelys semitestacea and Eunotosaurus africanus . Finally, we compare the dorsal rib histology of E. africanus to that of extinct and extant amniotes to determine if the highly modified hypaxial musculature used by modern turtles to ventilate their lungs was already present in E. africanus . These analyses indicate that the early stem-group turtle E. africanus has several turtle-specific lung ventilation characters. Our results place the origin of major portions of the unique lung ventilatory apparatus of extant turtles shortly after the divergence of the turtle stem lineage from those of other extant reptiles and approximately 50 million years before the oldest known fully developed shell. Our data indicate that as the dorsal ribs broadened over time they became more effective at supporting the trunk during locomotion but less effective for costal ventilation. Simultaneously, the hypaxial muscles were gradually freed from trunk support during locomotion and delegated purely to ventilating the lung. Thus, an easing of structural constraints through division of function (divergent specialization) between the dorsal ribs and the musculature of the body wall facilitated the evolution of both the novel turtle lung ventilation mechanism and the turtle shell. Homology of the respiratory muscles in turtles The body wall of amniotes is composed of a complex arrangement of muscles that are subdivided into epaxial and hypaxial groups [13] . We compared the hypaxial musculature from 55 turtle specimens from 24 species, whose phylogenetic distribution represents the diversity of crown turtles, with that of one tuatara, Sphenodon punctatus ( Fig. 2 and Supplementary Methods for list of specimens and taxa analysed). In most amniotes, the hypaxial muscles play a crucial role in respiration as well as in locomotion, which results in a mechanical conflict between these two functions [8] , [9] . Of the hypaxial muscles, which are divided into layers with different fibre orientations [13] , the M. obliquus abdominis and M. transversus abdominis are found in all turtles [14] and are active during lung ventilation [6] , [10] . Other hypaxial muscles, such as the Mm. intercostales , are reduced and eventually lost during embryonic ontogeny [7] . The general topography and innervation of the turtle M. obliquus abdominis and M. transversus abdominis are similar to those found in Sphenodon punctatus ( Fig. 2 and Supplementary Figs 1 and 2 ) and we agree with previous authors [6] , [10] , [14] on the homology of these muscles (see Table 1 and Supplementary Note 1 for a detailed discussion on the homology of each muscle used in respiration in turtles). However, the homology of the ‘M. diaphragmaticus,’ a name proposed by Bojanus [5] and used by subsequent authors [6] , [10] , [14] , is problematic. Unfortunately, muscles with identical names but doubtful homology have been described in turtles, mammals and crocodilians [6] thus confounding the evolutionary origin of the muscle in turtles. The M. diaphragmaticus of mammals and that of crocodilians are caudal to the lungs, whereas the ‘M. diaphragmaticus’ of turtles is cranial and ventral to the lungs, and there is widespread agreement that these muscles are not homologous across the three groups [2] . Rather the ‘M. diaphragmaticus’ of turtles shares several points of morphological identity with the M. transversus thoracis of other amniotes: (i) it has the same innervation (posterior (=ventral, see Supplementary Note 1 ) rami of the spinal nerves); (ii) it is positioned superficial to the peritoneum; (iii) it inserts into a tendinous aponeurosis that stretches over the entire width of the ventral peritoneum (as does the M. transversus abdominis posteriorly) and (iv) it originates from the ventral side of the cranial portion of the dorsal ribs (generally dorsal ribs two and three) [5] , [15] , [16] ( Fig. 2 and Supplementary Figs 1 and 2 ). Thus, we consider the ‘M. diaphragmaticus’ of turtles to be homologous to the amniote M. transversus thoracis (see Table 1 and Supplementary Note 1 ). Table 1 Primary respiratory muscles of turtles. Full size table Trunk skeleton of stem turtles We analysed the trunk anatomy of two early stem-group turtles, both of which have unfused ribs, by comparing them to extant turtles and a lepidosaur ( Fig. 3 and Supplementary Methods 1 for list of specimens and taxa analysed). The older E. africanus (Middle Permian, 260 mya) [4] , [17] , [18] , [19] , [20] shares several unambiguous derived characters with stem- and crown-group turtles, including paired gastralia and a greatly reduced trunk region (nine vertebrae) with nine pairs of broad and strongly curved dorsal ribs that are T-shaped in cross-section [4] , [17] , [18] , [19] , [20] ( Fig. 3a–c ). The ribs overlap sequentially and for the majority of their length ( Fig. 3b ). The rib heads are weakly bicapitate and articulate with the cranial half of the neural arch and the centrum, with the tuberculum and capitulum in a nearly vertical alignment [20] . This arrangement restricts costal movement to a cranio-caudal plane (bucket handle-like). The ribs have blunt and unfinished distal tips, indicating retention of cartilaginous ventral components ( Fig. 3d ). 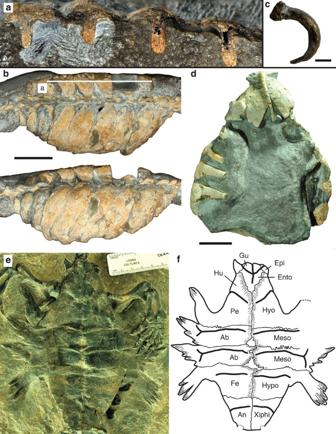Figure 3: The trunk anatomy of the early stem turtlesE. africanusandO. semitestacea. (a) Cross-section through dorsal ribs three to six along a natural break inE. africanusspecimen CM 86-341. (b) Two photographs ofE. africanusspecimen CM 86–341 in dorsolateral views showing how each rib overlaps the rib caudal to it for the majority of its length. White line marks ribs in part (a). Scale bar, 2 cm. (c) Right dorsal rib six ofE. africanusspecimen BP/I/4090 demonstrating the strong curvature of the dorsal ribs. Scale bar, 1 cm. (d) Ventral view ofE. africanusspecimen CM 777 that shows the unfinished and blunt to slightly concave distal tips of the dorsal ribs, indicating the presence of cartilaginous ventral components. Scale bar, 2 cm. (e,f) The plastron ofO. semitestacea(IVPP V13240) was covered in keratinous scutes (e) photograph and (f) line drawing exhibiting a pattern similar to that seen inP. quenstedti. Bold lines represent sulci between scutes and thin lines represent sutures between bones. Scute names are given on the left: Ab, abdominal scute; An, anal scute; Fe, femoral scute; Gu, gular scute; Hu, humeral scute; Pe, pectoral scute. Bone names are given on the right: Ento, entoplastron bone; Epi, epiplastron bone; Hyo, hyoplastron bone; Hypo, hypoplastron bone; Meso, mesoplastron bone; Xiphi, xiphiplastron bone. Figure 3: The trunk anatomy of the early stem turtles E. africanus and O. semitestacea. ( a ) Cross-section through dorsal ribs three to six along a natural break in E. africanus specimen CM 86-341. ( b ) Two photographs of E. africanus specimen CM 86–341 in dorsolateral views showing how each rib overlaps the rib caudal to it for the majority of its length. White line marks ribs in part ( a ). Scale bar, 2 cm. ( c ) Right dorsal rib six of E. africanus specimen BP/I/4090 demonstrating the strong curvature of the dorsal ribs. Scale bar, 1 cm. ( d ) Ventral view of E. africanus specimen CM 777 that shows the unfinished and blunt to slightly concave distal tips of the dorsal ribs, indicating the presence of cartilaginous ventral components. Scale bar, 2 cm. ( e , f ) The plastron of O. semitestacea (IVPP V13240) was covered in keratinous scutes ( e ) photograph and ( f ) line drawing exhibiting a pattern similar to that seen in P. quenstedti . Bold lines represent sulci between scutes and thin lines represent sutures between bones. Scute names are given on the left: Ab, abdominal scute; An, anal scute; Fe, femoral scute; Gu, gular scute; Hu, humeral scute; Pe, pectoral scute. Bone names are given on the right: Ento, entoplastron bone; Epi, epiplastron bone; Hyo, hyoplastron bone; Hypo, hypoplastron bone; Meso, mesoplastron bone; Xiphi, xiphiplastron bone. Full size image Like E. africanus , O. semitestacea (Late Triassic, 220 mya) [21] has nine cranio-caudally broadened ribs. Similar to crown turtles, the ribs are relatively straight (that is, less curved ventrolaterally), are single headed and have finished distal apices indicating loss of the ventral cartilages [4] , [21] . O. semitestacea has a fully developed plastron consisting of paired gastralia and dermal shoulder girdle bones (clavicles and interclavicle) similar to that found in crown turtles. The original morphological description by Li et al. [21] made no mention of scutes, that is, the keratinous plates that are found in all known extant and extinct shelled-turtles, with the exception of at least three groups that have secondarily lost them (represented by the extant Trionychidae, Carettochelys insculpta and Dermochelys coriacea ) [22] . Although turtle scutes are not usually preserved in the fossil record, they leave distinctive sulci on the dorsal surface of the shell that are readily observed in fossilized shell bones. Examination of the paratype of O. semitestacea (IVPP V13240) revealed the presence of such sulci on the plastron ( Fig. 3e,f ) forming a pattern similar to that of other stem turtles, including Proganochelys quenstedti [23] . The presence of sulci on the dorsal ribs could not be determined. However, of the three described O. semitestacea specimens, only two have dorsal portions of the ribs prepared. In addition, these two specimens (IVPP V15639, IVPP V15653) are not well-preserved relative to IVPP V13240, and the absence of sulci could reflect poor preservation rather than true morphology. There are currently no known turtles (crown or stem) that have scutes on the plastron but not the carapace (or vice versa). Amniote rib histology To determine if the highly modified hypaxial musculature ( Fig. 2 ) used by modern turtles to ventilate their lungs was present in E. africanus , we compared its dorsal rib histology based on 3 individuals (eight ribs in total) to that of 47 extinct and extant taxa representing all major amniote clades ( Supplementary Data 1 ). Sharpey’s fibres (ShFs), a component of the tendinous insertion of muscle into bone, can indicate the presence/absence of muscular attachments in extinct taxa [4] , [24] , [25] , [26] . All of the non-chelonian extant taxa examined ( N =36) possess intercostal muscles, and all of them exhibited ShF on both the cranial and caudal sides of the ribs ( Fig. 4 ). Most of the non-chelonian extinct taxa examined ( Supplementary Fig. 3a,b ) also preserved ShF on both the cranial and caudal sides of the ribs (also see Supplementary Fig. 4 ) including a pareiasaur ( Supplementary Fig. 3c–h ) from the same stratigraphic horizon as E. africanus and thus controlling for diagenetic alterations. Unfortunately, the rib histology from two broad ribbed parareptile taxa, Milleretta rubidgei and Pumilioparia pricei, was diagenetically altered such that the development and presence/absence of ShF could not be determined. A common snapping turtle ( Chelydra serpentina ; Fig. 5a ), which serves as a negative and positive control, lacked ShF where intercostal muscles have been lost and exhibited ShF where muscles are retained (for example, origin points of M. transversus; Fig. 5b–d ). 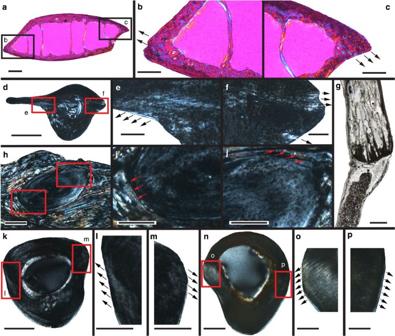Figure 4: Histology of extant amniote ribs. Histological sections of amniote ribs demonstrating the presence of Sharpey’s fibers (ShF) on both the cranial and caudal edges at the attachment sites of Mm. intercostales attachment sites. (a–c) Histological cross-section of a dorsal rib of a specimen (PIMUZ uncataloged) ofCapreolus capreolus(Mammalia) under polarized light with close-up images of the cranial (b) and caudal (c) edges of the rib. Scale bar, 1.0 mm inaand 500 μm inb,d. (d–f) Histological cross-section of a dorsal rib of a specimen (PIMUZ uncataloged) ofGavialis gangeticus(Archosauria) cross-polarized light (d; scale bar, 1.0 mm) with close-up images of the cranial (e) and caudal (f) edges of the rib. Scale bar, 125 μm ine,f. (g) Histological longitudinal section of the distal end of a dorsal rib of a specimen (PIMUZ uncataloged) ofA. mississipiensis(Archosauria) with calcified cartilage attached showing the blunt nature of the boney dorsal rib for attachment of ventral cartilaginous rib (compare withd). Scale bar, 1.0 mm. (h–j) Histological cross-section of gastralium of PIMUZ (uncatalogued specimen) ofA. mississipiensisembedded in abdominal musculature under cross-polarized light (h; scale bar, 500 μm) with close-up images of the cranial (i) and caudal (j) edges of the rib. Scale bar, 250 μm ini,j. (k–m) Histological cross-section of a dorsal rib of YPM 11160 (Corucia zebrata; Squamata) under cross-polarized (k; scale bar, 500 μm) light with close-up images of the cranial (l) and caudal (m) edges of the rib. Scale bar, 250 μm inl,m. (n–p) Histological cross-section of a dorsal rib of YPM11216 (Furcifer pardalis; Squamata) under cross-polarized (n; scale bar, 1 mm) light with close-up images of the cranial (o) and caudal (p) edges of the rib. Scale bar, 125 μm ino,p. Black and red arrows show where ShFs are visible. Figure 4: Histology of extant amniote ribs. Histological sections of amniote ribs demonstrating the presence of Sharpey’s fibers (ShF) on both the cranial and caudal edges at the attachment sites of Mm. intercostales attachment sites. ( a – c ) Histological cross-section of a dorsal rib of a specimen (PIMUZ uncataloged) of Capreolus capreolus (Mammalia) under polarized light with close-up images of the cranial ( b ) and caudal ( c ) edges of the rib. Scale bar, 1.0 mm in a and 500 μm in b , d . ( d – f ) Histological cross-section of a dorsal rib of a specimen (PIMUZ uncataloged) of Gavialis gangeticus (Archosauria) cross-polarized light ( d ; scale bar, 1.0 mm) with close-up images of the cranial ( e ) and caudal ( f ) edges of the rib. Scale bar, 125 μm in e , f . ( g ) Histological longitudinal section of the distal end of a dorsal rib of a specimen (PIMUZ uncataloged) of A. mississipiensis (Archosauria) with calcified cartilage attached showing the blunt nature of the boney dorsal rib for attachment of ventral cartilaginous rib (compare with d ). Scale bar, 1.0 mm. ( h – j ) Histological cross-section of gastralium of PIMUZ (uncatalogued specimen) of A. mississipiensis embedded in abdominal musculature under cross-polarized light ( h ; scale bar, 500 μm) with close-up images of the cranial ( i ) and caudal ( j ) edges of the rib. Scale bar, 250 μm in i , j . ( k – m ) Histological cross-section of a dorsal rib of YPM 11160 ( Corucia zebrata ; Squamata) under cross-polarized ( k ; scale bar, 500 μm) light with close-up images of the cranial ( l ) and caudal ( m ) edges of the rib. Scale bar, 250 μm in l , m . ( n – p ) Histological cross-section of a dorsal rib of YPM11216 ( Furcifer pardalis ; Squamata) under cross-polarized ( n ; scale bar, 1 mm) light with close-up images of the cranial ( o ) and caudal ( p ) edges of the rib. Scale bar, 125 μm in o , p . Black and red arrows show where ShFs are visible. 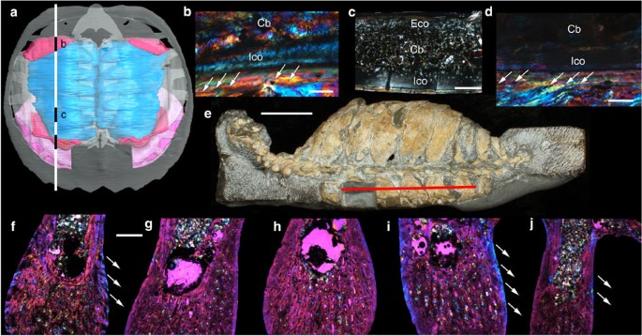Figure 5: Histological comparisons of the ribs of a crown turtle and the stem turtleE. africanus. (a) Three-dimensinal digital model of a crown turtle (C. serpentina) in dorsal view highlighting the shell, lungs (blue) and hypaxial muscles (red and pink). (b–d) Histological sections ofC. serpentina(USNM 324328) ribs taken along the length of the carapace (black/white line) show a modified connectivity of the M. transversus abdominis in which Sharpey’s fibres (ShF; white arrows) are present cranially (b; dorsal rib two, scale bar, 0.2 mm) and caudally (d; dorsal rib five, scale bar, 0.2 mm) but not in the other dorsal ribs (c; for example, three, six and so on, scale bar, 1 mm). (e–j) Histological sections ofE. africanus(CM86-341 (e), scale bar, 2 cm) (f–j) ribs taken along the length of the trunk (red line) show ShF (white arrows) on the caudal edge only of dorsal ribs three (f), six (i) and seven (j), but on neither edge of dorsal ribs four (g) and five (h). (f–j) Scale bar, 500 μm for each rib (f–j). Cb, cancellous bone; Eco, external cortex; Ico, internal cortex. Full size image Figure 5: Histological comparisons of the ribs of a crown turtle and the stem turtle E. africanus . ( a ) Three-dimensinal digital model of a crown turtle ( C. serpentina ) in dorsal view highlighting the shell, lungs (blue) and hypaxial muscles (red and pink). ( b – d ) Histological sections of C. serpentina (USNM 324328) ribs taken along the length of the carapace (black/white line) show a modified connectivity of the M. transversus abdominis in which Sharpey’s fibres (ShF; white arrows) are present cranially ( b ; dorsal rib two, scale bar, 0.2 mm) and caudally ( d ; dorsal rib five, scale bar, 0.2 mm) but not in the other dorsal ribs ( c ; for example, three, six and so on, scale bar, 1 mm). ( e – j ) Histological sections of E. africanus (CM86-341 ( e ), scale bar, 2 cm) ( f – j ) ribs taken along the length of the trunk (red line) show ShF (white arrows) on the caudal edge only of dorsal ribs three ( f ), six ( i ) and seven ( j ), but on neither edge of dorsal ribs four ( g ) and five ( h ). ( f – j ) Scale bar, 500 μm for each rib ( f – j ). Cb, cancellous bone; Eco, external cortex; Ico, internal cortex. Full size image Dorsal rib histology from three individuals (CM86-341 ribs 3–7 ( Fig. 5e–j ); NHM PV R 4949 rib 7; BP/1/7024 ribs 5-6 ( Supplementary Fig. 4 )) of E. africanus revealed that the cranial margins of all sampled ribs (3–7) lack ShF. ShFs are present along the caudal margins of dorsal ribs three ( Fig. 5f ), six ( Fig. 5i ) and seven ( Fig. 5j ) but not four and five ( Fig. 5g–h and Supplementary Fig. 4 ). The shortened trunk, cranio-caudally broadened dorsal ribs (each of which forms a strongly curved arch that overlaps the rib posterior to it for most of its length), and costovertebral articulations of E. africanus indicate a rigid trunk skeleton ( Fig. 3a–d ). The trunk of O. semitestacea was stiffened further by a fully ossified plastron covered with keratinous scutes ( Fig. 3e,f ). Such an inflexible body wall is ineffective for generating changes in intrapulmonary pressure [27] sufficient for ventilation, indicating that the plesiomorphic amniote costal ventilation mechanism was already abandoned in the most recent common ancestor of E. africanus and crown-group turtles. In addition, the lack of ShF on the cranial margins of dorsal ribs 3–7 ( Fig. 5 ) suggests the absence of intercostal muscles in E. africanus [4] . The inflexible trunk, combined with the loss of intercostal muscles in E. africanus [4] , indicates that costally mediated ventilation was replaced early in the turtle stem lineage. This situation presents two possibilities: either a fundamentally different ventilatory mechanism evolved and was later replaced by the one seen in crown turtles, or more parsimoniously, the mechanism in crown turtles was partially or fully developed in E. africanus and the last common ancestor that it shared with crown turtles. It is unlikely that early stem-group turtles relied upon gular or buccal pumping (ventilation effected by muscles of the mouth and/or throat), as this mode of breathing requires a large mouth-to-body size ratio [27] not present in E. africanus or O. semitestacea . Cutaneous respiration (including cloacal [28] and pharyngeal [29] , [30] , which supplements lung breathing in some modern turtles, is also unlikely, as it requires both permeable skin and an aquatic environment [31] . E. africanus , however, was terrestrial [19] and at least the plastron of O. semitestacea was covered by keratinous scutes ( Fig. 3e,f ). Rather, the histology of E. africanus provides strong evidence that part of the derived abdominal muscle-based lung-ventilation mechanism found in crown turtles was already in place early in the turtle stem lineage. In E. africanus , ShFs are present along the caudal margins of dorsal ribs three, six and seven but not four and five ( Fig. 5e–j ). The M. transversus of most modern turtles originates from ribs two and three, as well as ribs six and seven, but not in the mid-trunk (ribs four and five), where connections are present in non-chelonian amniotes ( Fig. 2 and Supplementary Figs 1 and 2 ). The remarkable correspondence of the ShF pattern between E. africanus ( Fig. 5e–j ) and crown turtles ( Fig. 5a–d ) supports the hypothesis that the derived muscular sling, formed by the M. transversus and used by modern turtles to expire, was already present in this Middle Permian form. Unlike the M. transversus, strong osteological correlates for the derived hypaxial muscle used in turtle inspiration, the M. obliquus abdominis, do not exist and the inverted dome-like morphology found in crown turtles cannot be established in E. africanus . However, ancestrally the M. obliquus extends between the pelvic and shoulder girdles attaching to each dorsal rib via tendinous sheets, as in Sphenodon punctatus ( Fig. 2d ). The absence of ShF on dorsal ribs four and five indicates these plesiomorphic connections were not present in E. africanus so that perhaps the modified arrangement of this muscle seen in extant turtles was also present in this early stem turtle. The connection of the M. obliquus with the gastralia is unknown, so it is not possible to determine if they supported an inverted, cup-shaped M. obliquus, which powers active inspiration in crown turtles. In addition, if ShFs are found in the gastralia of E. africanus , it would not be possible to determine if they represent the M. obliquus or other abdominal muscles (for example, M. rectus) that also have their origination and/or insertion points here [32] . Active inspiration in E. africanus was likely not primarily driven by the broadened dorsal ribs as they create a largely rigid body wall and furthermore, the intercostal muscles used to actively move the ribs to create volumetric changes in the coelomic cavity are lacking. However, the dorsal ribs are not sutured together, as in crown turtles, and limited movement was possible, indicating that some costal ventilation may have been possible. This costal ventilation may have been effected by the cartilaginous ventral ribs known to be present in E. africanus ( Fig. 3d ). Such a duplication of inspiratory function (ribs and hypaxial muscles) in E. africanus would allow for subsequent specialization of the M. obliquus and eventually further specialization of the ribs and gastralia, which are the primary shell elements in crown turtles. In addition, passive inspiration was likely possible in the terrestrial E. africanus and may have helped facilitate the transition in active inspiration from the ancestral state involving both the intercostal and hypaxial (abdominal) muscles to the highly derived hypaxial muscle-based mechanism found in turtles. Whereas active inspiration in turtles is effected by hypaxial musculature (mainly the M. obliquus abdominis), experimental data on snapping turtles ( C. serpentina ) indicate that inspiration can occur passively on land, via a gravity-based mechanism [6] . Specifically, the reduced plastron of C. serpentina provides only limited support for the weight of the viscera on land, where the buoyant force of water does not offset gravity. The viscera, part of which are attached to the ventral portion of the lungs ( Fig. 6 ), were shown experimentally to passively pull downward on the latter, particularly after they have been lifted dorsally during expiration [6] . Dorsal attachment to the shell ( Fig. 6 ) prevents the entire lung from being pulled ventrally. Rather, only the ventral portion moves, increasing the volume of the pliable lung, thereby reducing intrapulmonary pressure and affecting inspiration. 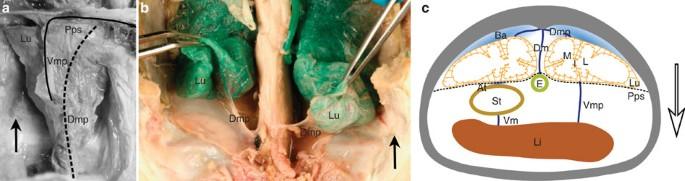Figure 6: The coelomic connections of the lungs in turtles. (a) Right lung (Lu) of a specimen (ZMB uncatalogued; carapace length=270 mm) ofC. serpentinain ventral view indicating the course of the dorsal (Dmp) and ventral (Vmp) mesopneumonia. Modified after Lambertzet al.15(b) Both lungs of a wet specimen ofTrachemys scripta(Rheinische Friedrich-Wilhelms-Universität Bonn uncatalogued; carapace length=170 mm) in ventral view showing the dorsal mesopneumonia. Modified after Lambertz and Perry48. (c) Schematized cross-section through the trunk of a turtle in caudal view. The lungs are suspended dorsally via either the dorsal mesopneumonia or a broadened attachment (Ba). The liver (Li) attaches directly to the right lung via the ventral mesopneumonium and indirectly to the left lung via the ventral mesentery (Vm) through the stomach (St), which is broadly attached (At) to the left lung. A postpulmonary septum (Pps) is present to varying degrees of completeness and provides further support for the lungs. Gravity (white arrow) acting on the viscera, particularly the liver, can expand the lungs and passively generate inspiratory airflow. E, esophagus; Dm, dorsal mesentery; I, intrapulmonary bronchus; L, lateral chamber of the lung; M, medial chamber of the lung. Figure (c) modified from Gräper35. Figure 6: The coelomic connections of the lungs in turtles. ( a ) Right lung (Lu) of a specimen (ZMB uncatalogued; carapace length=270 mm) of C. serpentina in ventral view indicating the course of the dorsal (Dmp) and ventral (Vmp) mesopneumonia. Modified after Lambertz et al. [15] ( b ) Both lungs of a wet specimen of Trachemys scripta (Rheinische Friedrich-Wilhelms-Universität Bonn uncatalogued; carapace length=170 mm) in ventral view showing the dorsal mesopneumonia. Modified after Lambertz and Perry [48] . ( c ) Schematized cross-section through the trunk of a turtle in caudal view. The lungs are suspended dorsally via either the dorsal mesopneumonia or a broadened attachment (Ba). The liver (Li) attaches directly to the right lung via the ventral mesopneumonium and indirectly to the left lung via the ventral mesentery (Vm) through the stomach (St), which is broadly attached (At) to the left lung. A postpulmonary septum (Pps) is present to varying degrees of completeness and provides further support for the lungs. Gravity (white arrow) acting on the viscera, particularly the liver, can expand the lungs and passively generate inspiratory airflow. E, esophagus; Dm, dorsal mesentery; I, intrapulmonary bronchus; L, lateral chamber of the lung; M, medial chamber of the lung. Figure ( c ) modified from Gräper [35] . Full size image To better understand passive inspiration mechanism in turtles, it is necessary to consider their pulmonary anatomy and how the lungs are situated in the coelomic cavity. The lungs of all turtles are multi-chambered, with individual chambers branching off from a central intrapulmonary bronchus in a hierarchical sequence [33] . Plesiomorphically, there is a row of larger lateral and smaller medial chambers ( Fig. 6c ). The intrapulmonary bronchus thus lies closer to the vertebral axis of the animal than does the sagittal midline of the lung ( Fig. 6c ). Dorsally, the visceral pleura adhering to the surface of the lungs connects to the parietal pleura either via discrete mesopneumonia or through a broadened attachment [34] ( Fig. 6 ). When dorsal mesopneumonia are present, they are situated over the portion of the lung that houses the intrapulmonary bronchus, thus providing mechanical stabilization for this central conductive structure ( Fig. 6 ). Such an anatomical configuration forces the central intrapulmonary airway, which has additional cartilage reinforcements in most taxa [35] , to be open at all times. In addition to these dorsal connections, the lungs are connected to other viscera on their ventral surfaces ( Fig. 6 ). In most turtles, the right lung attaches via the ventral mesopneumonium directly to the liver. Cranially, the left lung is broadly attached to the stomach, which in turn is connected to the liver via the ventral mesentery ( Fig. 6 ). In both cases, the ventral connections coincide closely with the course of the central intrapulmonary bronchus. A gravity induced pull of the liver hence acts indirectly (via the various inter-organ connections) on the relatively immobile regions of the lung. This passive gravitational mechanism can thereby achieve an opening of the airways combined with a reduction in intrapulmonary pressure, resulting in inspiration. A similar passive inspiratory mechanism is plausible in terrestrial E. africanus , whose ventral trunk skeleton consists of paired gastralia [4] , which, like the slender plastron found in C. serpentina , provide a lesser degree of support for the weight of the viscera on land––particularly after lifting of the viscera by the contraction of the sling-like M. transversus –– than found in a turtle with a more robust plastron. Given the coelomic integration of the lungs among extant amniotes, and turtles in particular [15] , [36] , [37] , [38] , we can infer a similar set of inter-organ connections for E. africanus . The gravity-induced ventral pull of the viscera would passively open the lungs, as documented in C. serpentina on land, and increase the volume of the pliable lung, resulting in lower intrapulmonary pressures and passive inspiration. Even though the actual nature of the M. obliquus abdominis cannot be reconstructed with certainty for E. africanus or any other extinct stem group representative of turtles (see above), our functional approximation of its respiratory apparatus allows us to recognize this passive mode of inspiration as a plausible alternative or at least additional solution, which serves as a minimum explanation for how the animal could have supplied its metabolic demand for oxygen. Our findings suggest that the early stem lineage of turtles (at least as early as E. africanus ) deviated from the basal amniote body plan (in which locomotion and breathing are coupled) and evolved a division of function in which the ribs took on a stabilizing role, whereas the abdominal muscles became specialized to ventilate the lungs ( Fig. 7 ). The plausibility of this scenario is bolstered by a similar, albeit less extreme, division of labour among broad-ribbed mammals (for example, the anteater Cyclopes didactylus ; the loris Arctocebus calabarensis ; the tree shrew Ptilocercus lowii ) [39] . As the ribs of early stem turtles began to broaden and overlap, they became more effective at stabilizing the trunk ( Fig. 7 ) but less effective contributors to pulmonary ventilation. This shift liberated the M. transversus, M. obliquus and Mm. intercostales from their functions in trunk stabilization, allowing them either to specialize for ventilation (M. transversus and M. obliquus) or to be lost (Mm. Intercostales; Fig. 3 ). Once ventilation no longer required flexibility of the trunk, a constraint on the dorsal ribs was removed, allowing them to further broaden, fuse and eventually form a rigid carapace, as seen in turtles more crownward than Odontochelys . This model, which is based on an easing of structural constraints through a division of function (divergent specialization), places the origin of the unique lung ventilatory apparatus of extant turtles shortly after the divergence of turtles from other reptiles, well within the Paleozoic and at least 50 million years before the oldest known fully developed shell, from the Late Triassic (Middle Norian, Proterochersis robusta ) [40] . 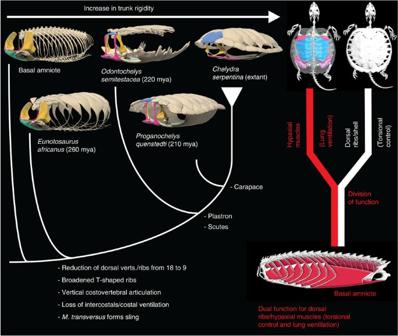Figure 7: Evolutionary scenario for the origin of the unique lung ventilation apparatus of turtles. Phylogeny (left) of stem turtles4,17showing increasing trunk rigidity towards the crown (Note: the plastron is formed by the fusion of gastralia, interclavicle and clavicles, whereas the carapace is formed by the fusion of ribs, vertebrae, cleithra and ossified osteoderms found along the perimeter of the shell)49. Our results suggest that the early stem lineage of turtles evolved a division of function in which the dorsal ribs took on a purely stabilizing role, whereas abdominal muscles became specialized for ventilating the lungs (right). Homology of the shoulder girdle elements follows Lysonet al.49Basal amniote redrawn and modified from Carrier50. Clavicle: pink; cleithrum: blue; interclavicle: green; scapula: yellow. Figure 7: Evolutionary scenario for the origin of the unique lung ventilation apparatus of turtles. Phylogeny (left) of stem turtles [4] , [17] showing increasing trunk rigidity towards the crown (Note: the plastron is formed by the fusion of gastralia, interclavicle and clavicles, whereas the carapace is formed by the fusion of ribs, vertebrae, cleithra and ossified osteoderms found along the perimeter of the shell) [49] . Our results suggest that the early stem lineage of turtles evolved a division of function in which the dorsal ribs took on a purely stabilizing role, whereas abdominal muscles became specialized for ventilating the lungs (right). Homology of the shoulder girdle elements follows Lyson et al. [49] Basal amniote redrawn and modified from Carrier [50] . Clavicle: pink; cleithrum: blue; interclavicle: green; scapula: yellow. Full size image Material analysed The hypaxial musculature from 55 turtle specimens from 24 species, whose phylogenetic distribution covers the basal divergence within crown turtles, was dissected and compared with that of one tuatara, Sphenodon punctatus ( Supplementary Methods 1 for list of specimens analysed). The skeletal morphology from the trunk region from 37 E. africanus and 3 O. semitestacea specimens was examined ( Supplementary Methods 1 for list of specimens analysed). Eight dorsal ribs from three E. africanus specimens were sectioned for histology and compared with that of 46 extinct and extant taxa representing all major amniote clades ( Supplementary Data 1 ). In addition, two C. serpentina carapaces were sectioned for histology ( Supplementary Data 1 ). Specimens of C. serpentina (deceased), Varanus exanthematicus (live) , Alligator mississippiensis (live) and Gallus domesticus (deceased) were imaged using computed tomography (CT). Histology The petrographic thin sections (see Supplementary Data 1 for list of taxa) were prepared using standard procedures [41] and analysed using a LEICA DM 2500 M composite microscope, equipped with a LEICA DFC420 C digital camera and Nikon Eclipse 50i Polarizing microscope, equipped with a DS-Fi1 digital camera. Processing and preparation of images was accomplished using Adobe Photoshop and Illustrator, and CorelDraw. The description of histological structures follows Francillon-Vieillot et al. [42] and Sanchez et al. [25] for recognition of entheses and extrinsic fibres within the bone. Sharpey’s fibres are herein identified as conspicuous fibres and coarser fibre bundles that extend obliquely into the cortical periosteally deposited bone tissue. In cross-polarized light (and cross-polarized light using a lambda compensator), these appear as fibre bundles that show different extinction patterns compared with the surrounding bone tissue because of different fibre orientation. Computed tomography The CT scans were performed at the University of Utah South Jordan Medical Center in accordance with and approved by the University of Utah Institutional Animal Care and Use Committee. Live unsedated animals (subadult V. exanthematicus (female) and subadult A. mississippiensis (sex unknown)) were scanned during a natural apnea; deceased specimens (adult G. domesticus (female) and adult C. serpentina (sex unknown)) were intubated and the lungs artificially inflated by hand with a 60-cc syringe. The individuals were CT scanned at 100 kVp and 400 MA with a slice thickness of 0.6 mm at intervals of 0.4 mm (with 0.2 mm overlap). Three-dimensional digital models were segmented in Avizo version 7.1 ( http://www.vsg3d.com/avizo/standard ) by hand, using a Wacom Intuos4 pen tablet. The images were edited and modified into figures in Adobe Photoshop. How to cite this article : Lyson, T. R. et al. Origin of the unique ventilatory apparatus of turtles. Nat. Commun. 5:5211 doi: 10.1038/ncomms6211 (2014).